Redox chemistry and metal–insulator transitions intertwined in a nano-porous material Metal-organic frameworks are nano-porous adsorbents of relevance to gas separation and catalysis, and separation of oxygen from air is essential to diverse industrial applications. The ferrous salt of 2,5-dihydroxy-terephthalic acid, a metal-organic framework of the MOF74 family, can selectively adsorb oxygen in a manner that defies the classical picture: adsorption sites either do or do not share electrons over a long range. Here we propose, and then justify phenomenologically and computationally, a mechanism. Charge-transfer-mediated adsorption of electron acceptor oxygen molecules in the metal-organic framework, which is a quasi-one-dimensional electron-donor semiconductor, drives and is driven by quasi-one-dimensional metal–insulator–metal transitions that localize or delocalize the quasi-one-dimensional electrons. This mechanism agrees with the empirical evidence, and predicts a class of nano-porous semiconductors or metals and potential adsorbents and catalysts in which chemistry and metal–insulator–metal transitions intertwine. Most adsorbents—materials essential to chemical industry—are porous solids of high surface area [1] . Metal-organic frameworks (MOFs) [2] , [3] , [4] is a vast and rapidly expanding class of synthetic adsorbents. MOFs find applications in gas separation [5] and storage [6] , [7] , [8] , just as do their prototypes, zeolites. The geometry of a MOF interconnects the metal cations and ligands (linkers) in a three-dimensional nano-porous lattice. The vertices of the lattice are the metal cations and its bridges are the linkers. If the cations are redox-labile transition metals, the MOF can participate in electron transfer-driven (that is redox) chemistry [9] , [10] , [11] , unlike the redox-rigid zeolites. Separation of O 2 from air [12] , [13] is an indispensable step in industrial applications [14] . Since O 2 is the only major prominent redox-labile component in dry and clean air [15] , a separation strategy can rely on differences between adsorption of the redox-rigid gases and O 2 over a redox-labile adsorbent [9] , [11] , [16] . Fe 2 (DOBDC), the ferrous salt of 2,5-dihydroxy-terephthalic acid H 4 DOBDC ( Fig. 1a ), is a MOF of the MOF74 family ( Fig. 1e ) and is also a redox-active adsorbent whose reactive exposed Fe sites [17] selectively bind O 2 [9] ( Fig. 1d , inset). In particular, Fe 2 (DOBDC) is an adsorbent suitable for O 2 separation at temperatures . However, the material adsorbs O 2 irreversibly within the pressure range of ref. 9 and above the temperature T A , which is below the temperatures that are desirable in the industrial separation applications [9] . 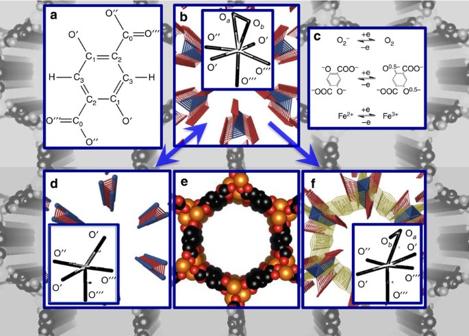Figure 1: Oxygen adsorption in the MOF74. (a) The geometry of the linker DOBDC. (c) Charge transfer channels in the MOF74. (e) The geometry of the MOF74. The linker’s carbons and hydrogens are black, the linker’s oxygens are red and the metal ions are orange. The metal ions around the third-order twist axises occupy general position sites. The chirality of the adjacent metal chains is opposite. The linker occupies the centres of the symmetry positions. (b,d,f) The connectivity of the charge flow in π-O2, Fe2(DOBDC) andσ-O2, respectively; the blue colour encodes flow at the energies, while the purple or yellow colours encode a higher energy flow. (b,d,f) (insets) The first coordination sphere of the metal site in π-O2, Fe2(DOBDC) and σ-O2, respectively; O2in π-O2is aligned along the O′′–O′′′ direction. Figure 1: Oxygen adsorption in the MOF74. ( a ) The geometry of the linker DOBDC. ( c ) Charge transfer channels in the MOF74. ( e ) The geometry of the MOF74. The linker’s carbons and hydrogens are black, the linker’s oxygens are red and the metal ions are orange. The metal ions around the third-order twist axises occupy general position sites. The chirality of the adjacent metal chains is opposite. The linker occupies the centres of the symmetry positions. ( b , d , f ) The connectivity of the charge flow in π-O 2 , Fe 2 (DOBDC) and σ -O 2 , respectively; the blue colour encodes flow at the energies , while the purple or yellow colours encode a higher energy flow. ( b , d , f ) (insets) The first coordination sphere of the metal site in π-O 2 , Fe 2 (DOBDC) and σ-O 2 , respectively; O 2 in π-O 2 is aligned along the O′′–O′′′ direction. Full size image Reference [9] 9 establishes experimentally an atypical pattern of O 2 adsorption in Fe 2 (DOBDC) that has neither been previously seen nor understood in the MOF chemistry. O 2 chemisorbs in Fe 2 (DOBDC) in the form of a superoxide adduct, (DOBDC) for 0≤ x ≤1 (to be denoted π-O 2(1− x ) ), at the temperatures , and the type of structure of the MOF remains intact under an O 2 load. The π-O 2(1− x ) fully desorbs its O 2 and regenerates back into Fe 2 (DOBDC) on lowering the O 2 partial pressure at . Remarkably, π-O 2(1− x ) converts exothermically at T ≈ T A to the peroxide adduct, (DOBDC) for (to be denoted σ -O 2(1− x ) ), while losing about half of its O 2 . As such, σ -O 2(1− x ) neither desorbs nor chemisorbs O 2 . The O 2 coordinates the exposed Fe site symmetrically in π-O 2(1− x ) ( Fig. 1b , inset) but asymmetrically in σ-O 2(1− x ) ( Fig. 1f , inset). The experimental structural data at low temperatures [9] indicate that no more than one O 2 molecule per a metal site chemisorbs immediately at an Fe site at the distance about 2 Å away and the O–O bonds elongate, and, if any additional O 2 molecules physisorb, they remain at least twice as far away from an Fe site and their O–O bonds remain as long as that in a free O 2 . The green-coloured semiconductor Fe 2 (DOBDC) has the apparent band gap of about 0.5 eV but Mössbauer spectroscopy [9] suggests that the black π-O 2(1− x ) is a mixed-valence compound whose Fe II–III sites are identical, that is, it appears to be a metal. In contrast, Fe 2 (DOBDC) remains a semiconductor on adsorption of the redox-rigid N 2 , and physisorption of O 2 or N 2 in the homologous Zn 2 (DOBDC) does not affect its optical response at visible wavelengths. These experiments suggest that the distributed and intermittent flow of the electrons along the MOF must play a crucial role during the adsorption of O 2 in the redox-labile Fe 2 (DOBDC) but not in the redox-rigid Zn 2 (DOBDC). Unlike the redox properties, the geometries of these materials [9] , [18] are nearly identical. Hence, the differences in their redox properties must originate in the electronic structure—the other side of the material’s chemical identity. This report shows that O 2 adsorption in Fe 2 (DOBDC) is quite an unusual (but likely not uncommon) redox chemical reaction for nano-porous materials. It is often taken for granted that charge transfer confined to the individual adsorption sites controls redox chemistry of nano-porous materials. It turns out that Fe 2 (DOBDC) is a strongly correlated quasi-one-dimensional (1D) material that undergoes a sequence of metal–insulator–metal transitions intertwined with O 2 adsorption-desorption, and the charge transfer during O 2 adsorption-desorption in Fe 2 (DOBDC) involves cooperation of many interconnected adsorption sites rather than a single site. The parameter T A controls the activation barrier for this process. To the best of our knowledge, this report is the first description of this type of redox chemistry in nano-porous materials. Metal–insulator transitions and adsorption-desorption The MOF Fe 2 (DOBDC), as a nano-porous material, is a sponge of a definite geometry and maximal porosity. The MOF’s geometry defines the boundary that delimits two dual regions: the network of the pores where the adsorbate can flow and the space where the electrons and atoms of the MOF concentrate. As the electron acceptors O 2 [19] adsorb from or desorb into the pores and the electrons flow out or into the MOF, the charge can flow along the boundary of the MOF ( Fig. 1e ) according to the likelihoods of the formal redox events that connect distinct sites and involve the metal or the linker as Fig. 1c explains. Because of possible metal–insulator transitions, the charge flow can fracture into or reconnect from disconnected null dimensional atom-like, one-dimensional chain-like and two dimensional surface-like conducting components within the geometry of the MOF during adsorption of O 2 . Since the properties of metals, insulators and metal–insulator transitions differ qualitatively in null, one or higher dimensions [20] , so must redox chemistry, as the chemistry of charge flow. It remains to be shown that the processes in Fig. 1b,d,f (insets) constrain the changes in the charge distribution during O 2 adsorption to these in Fig. 1b,d,f , and that the consequences of these constraints are consistent with the empirical evidence of ref. 9 . A model and its validation To arrive at and validate a model of O 2 adsorption, this report relies on quantum chemistry calculations as detailed in Methods section. The total energy, the geometries, the harmonic vibrational frequencies and the electronic band structure are modelled within the numerical spin-unrestricted density functional theory (DFT) using the PW91+U approximation to the exchange-correlation energy as implemented in refs 21 , 22 and as further detailed in Methods section (Density functional theory calculations). The optical absorption spectrum of ref. 9 is interpreted in terms of a model crystal field Hamiltonian and the PW91+U method as detailed in Methods sections (Density functional theory calculations and Crystal field Hamiltonian: top-down approach). The low-lying excited states of Fe 2+ and [Fe−O 2 ] 2+ in the midst of the crystal field are computed in the CIS(D), state-averaged CASSCF MP2, and TD-DFT approximations as implemented in ref. 22 and as detailed in Methods section (Crystal field Hamiltonian: bottom-up approach). The electron correlation effects in the extended system beyond the PW91+U level of theory are treated within the density matrix renormalization group (DMRG) [23] method as implemented in ref. 24 and as detailed in Methods sections (Model of interacting electrons and DMRG calculations). The model geometries of Fe 2 (DOBDC) and π-O 2 , which are computed with PW91+U at U =0, are enclosed in Supplementary Data 1 and 2 . As Table 1 shows, the model geometries agree with the experimental data at a level no worse than 0.3 and 0.1 Å, respectively. The computed and experimental band gaps in Fe 2 (DOBDC) are matched, and the computed optical excitation energies also agree with the experiment [9] . Since the PW91+U band structure theory at U =0 underestimates the electron–electron interaction in the strongly correlated semiconductor Fe 2 (DOBDC), it also underestimates the band gap. As U increases, the band gap increases achieving the empirical value of about 0.5 eV at the repulsion U of about 0.5 eV ( Supplementary Fig. 1 ). Since the band structure of Fe 2 (DOBDC) at U =0 is gapless in contradiction with the experiment, but the gap opens on introduction of the electron–electron repulsion U =0.5 eV, it exemplifies a correlated insulator. The computed binding energy of −0.56 eV of O 2 in π-O 2 also agrees satisfactorily with the experimental saturation heat of adsorption at −0.68 eV. The binding of O 2 in π-O 2 in the O–O bond-down configuration is more favourable than in the end-down configuration (by 0.3 eV), which is consistent with the experiment. The self-consistent magnetic structure features the absolute magnetization of 4.1μ B per Fe and the total magnetization of zero, which is consistent with the experiment assuming that the single-ion anisotropy effects at the Fe sites are neglected [7] , [9] . Table 1 The structural parameters of M 2 (DOBDC), π -O 2 , σ -O 2 and the linker. Full size table The electron flow is low dimensional To establish that the electrons flow from Fe 2 (DOBDC) to O 2 during adsorption, it is sufficient to recognize that the elongation of the O–O bonds signals the electron transfer to O 2 [25] , and the O–O bonds, computed and experimental in π-O 2 and experimental in σ -O 2 , [9] are longer than the bond in the free O 2 by 0.09(0.05) and 0.4 Å, respectively. 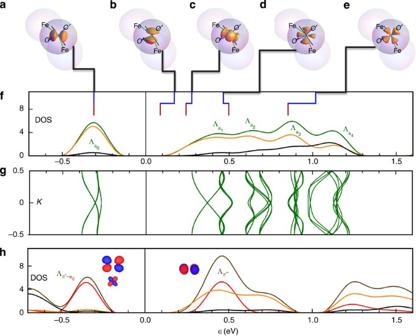Figure 2: The electronic structure of the MOF74. (a–e) The shapes of the electron distribution in the crystal field states5A0,5A1,5A2,5A3,5A4at an Fe2+site, respectively. (f) The PW91+U density of states (DOS) in Fe2(DOBDC) atU=0.5 eV (solid green). The upper (blue) and lower (red) vertical bars denote the energy levels that are determined using the top-down and bottom-up approaches, respectively. (g) The PW91+U band structure along the trigonal direction (κ) for Fe2(DOBDC). The Fermi level corresponds to ?=0 eV so that the states with ?<0 are doubly occupied. Each of the fived-orbitalsa0,1,2,3,4at the three translationally distinct metal sites in the unit cell of the 1D helical chain (Fig. 1e) gives rise to a triplet of the bands, which has an appearance of a ‘swallow’s tail’. (h) The PW91+U DOS in π-O2(solid brown) atU=0.5 eV; the inset shows the π′–a0antibonding and π′′ nonbonding orbitals. Inf,h, the orange, red and black lines denote projected densities of states on the 3datomic orbitals of the iron, 2patomic orbitals of the adsorbed oxygen, and the 2sand 2patomic orbitals of the oxygen and carbon in the DOBDC, respectively. The DFT calculations further corroborate that every O 2 in π-O 2 hosts 0.44 e excess electrons ( Table 2 ). Table 2 The Bader charges in units of the elementary charge. Full size table If the electrons flow to an O 2 , then this flow originates from the Fe site just underneath it. To elucidate the mechanism underlying this flow, the following model is considered. If the intersite electron flow is discarded, then the effect of the Fe 2 (DOBDC) crystal on the Fe site is that of a polarizing crystal field. A numerical density functional theory estimates this crystal field. For the strongly correlated redox-labile Fe site in the presence of the polarizing crystal field, the bottom-up wavefunction-based quantum chemistry (Methods Section (Crystal field Hamiltonian: bottom-up approach)) predicts the energy levels as well as the shapes of the electronic distributions in these levels. In contrast, the experimental optical absorption spectrum and geometry [9] constrain in a top-down approach the form of and the values of the adjustable parameters within the crystal-field Hamiltonian (Methods Section (Crystal field Hamiltonian: top-down approach)). The electronic states that are obtained by the bottom-up and top-down approaches agree at the Fe site in Fe 2 (DOBDC) as shown in Fig. 2f ; Supplementary Fig. 2 . The lowest excitations that are centered at an Fe site occur between the ground 5 A 0 and the excited 5 A 1 , 5 A 2 , 5 A 3 and 5 A 4 crystal field multiplets ( Fig. 2a–e ), which descend from the ground state multiplet 3 d 6 5 D of the free Fe 2+ . Figure 2: The electronic structure of the MOF74. ( a – e ) The shapes of the electron distribution in the crystal field states 5 A 0 , 5 A 1 , 5 A 2 , 5 A 3 , 5 A 4 at an Fe 2+ site, respectively. ( f ) The PW91+U density of states (DOS) in Fe 2 (DOBDC) at U =0.5 eV (solid green). The upper (blue) and lower (red) vertical bars denote the energy levels that are determined using the top-down and bottom-up approaches, respectively. ( g ) The PW91+U band structure along the trigonal direction (κ) for Fe 2 (DOBDC). The Fermi level corresponds to ?=0 eV so that the states with ?<0 are doubly occupied. Each of the five d -orbitals a 0,1,2,3,4 at the three translationally distinct metal sites in the unit cell of the 1D helical chain ( Fig. 1e ) gives rise to a triplet of the bands, which has an appearance of a ‘swallow’s tail’. ( h ) The PW91+U DOS in π-O 2 (solid brown) at U =0.5 eV; the inset shows the π′– a 0 antibonding and π′′ nonbonding orbitals. In f , h , the orange, red and black lines denote projected densities of states on the 3 d atomic orbitals of the iron, 2 p atomic orbitals of the adsorbed oxygen, and the 2 s and 2 p atomic orbitals of the oxygen and carbon in the DOBDC, respectively. Full size image In [Fe−O 2 ] 2+ in the crystal field, the electron-acceptor antibonding molecular orbital π g of O 2 splits into the components π′ and π′′ (out and in the plane of the adsorption site), and π′ and the electron-donor molecular orbital a 0 match in shape ( Fig. 2a,h ). The ground and first excited states of an [Fe−O 2 ] 2+ site at the geometry of π-O 2 are and , respectively. The first excitation energy is about 1 eV (see Supplementary Table 1 ). For the PW91+U model for the extended system π-O 2 ( Fig. 2f,h ), the projected densities of electronic states on the valence 3 d orbitals of Fe and 2 p orbitals of O in O 2 further elucidate the nature of the Fe–O 2 chemisorption bond. The molecular orbitals π′ and π′′ at O 2 form bonding and antibonding combinations with the a 0,1,2,3,4 orbitals at the Fe site so that all the bonding orbitals and some antibonding orbitals are occupied. As O 2 adsorbs, the initial high density of the occupied 3 d -like states of Fe ( Fig. 2f ) decreases, while the density of the 2 p -derived states at O 2 increases ( Fig. 2h ) just below the Fermi level. The donation-backdonation three-centre bond between O 2 and Fe forms in the direction of the overlap between a 0 and π′, and during adsorption the electrons flow from a 0 at Fe to π′ at O 2 . The binding of O 2 in π-O 2 is reminiscent to that of ethylene in donation-backdonation π-complexes [26] . In fact, the ground states of the dioxygen and ethylene, and 1 A g H 2 C=CH 2 , are equivalent through a deformation that fuses the protons of the ethylene into their neighboring carbon nuclei. This analogy reflects the observation of the π-complexes [7] , [9] in Fe 2 (DOBDC). If electrons flow from the Fe underneath the O 2 , then this flow can originate from an adjacent Fe site within the 1D chain of Fe sites or from an adjacent 1D chain of Fe sites through the linker ( Fig. 1c ). To examine these possibilities, the electronic band structure is calculated using a PW91+U method (Methods section (Density functional theory calculations)). Every crystal field multiplet 5 A 0,1,2,3,4 corresponds to a triple Λ a 0 , 1 , 2 , 3 , 4 of a 0,1,2,3,4 -like electronic bands ( Fig. 2g ) in the semiconductor Fe II (DOBDC), while the antibonding combinations of a 0 and π′ define the valence band in π-O 2 ( Fig. 2f,h ). The dispersion within and the splitting of these bands quantify the extent and direction of the electron delocalization upon excitations. The bands Λ a 0 , 1 , 2 are dispersionless away from the trigonal direction, and their hybridization with the DOBDC-centred electronic states is negligible, while the couplings of the bands along the adjacent metal ion chains are two orders of magnitude smaller than the widths of the bands themselves; the interchain coupling is particularly small for the states surrounding the Fermi level. Therefore, the electrons in these bands are 1D along the parallel 1D metal ion chains in the trigonal direction ( Fig. 1d ). More pronounced deviations from the 1D character arise at the energy scale around 1.1 eV of the Λ a 3 , 4 bands, which hybridize through the linker; the deviation is also present to a much lesser degree in the other bands away from the Fermi level. The valence bands in π-O 2 are 1D along the trigonal direction around the Fermi level ( Fig. 1b ). The lowest electronic excitations in π-O 2(1− x ) in the band structure picture are intersite excitations that involve the partially filled Λ a 0 − π ′ bands rather than the intrasite excitations. The projected density of states on valence orbitals of the DOBDC further suggests that the coupling through the linker is very small in Fe 2 (DOBDC) and in π-O 2 at the energies just below the Fermi level where the band Λ a 0 is concentrated ( Fig. 2h ), but the states of the DOBDC become involved if the band Λ a 0 is sufficiently depleted of its electrons. The trends in the geometry of the linker further suggest that the electrons do not flow along the linker in Fe 2 (DOBDC) and π-O 2 ( Fig. 1b,d ), but the electrons must flow along the linker during conversion of π-O 2 to σ -O 2 ( Fig. 1f ). The formal anion DOBDC 4− , as a 2,5-quinolate anion, is a reducer. Its prototype, the 2,5-benzene quinolate, is the active agent in the reductive developers in the silver halide photography due to the capacity to transfer electrons from Ag 0 to nearby Ag + (ref. 27 ). Similarly, DOBDC 4− may oxidize ( Fig. 1c ) while transferring the electrons between the Fe sites in the adjacent chains. An indicator of the involvement of the DOBDC is the shortening of the C 1 –O′ and C 2 –C 3 bonds ( Fig. 1a ). This distortion is ruled out ( Table 1 ) at a level no worse than 0.03 Å in the redox rigid Mg 2 (DOBDC) and Zn 2 (DOBDC) as well as in Fe 2 (DOBDC) and π-O 2 . However, the distortion is manifest in σ-O 2(1− x ) . Indeed, Table 1 shows that those bond lengths of the free reduced form of the ligand DOBDC 4− , which are meant to transfer (C 1 –C 2 , C 2 –C 3 , C 3 –C 1 , C 1 –O′), do transfer to the redox unremarkable Mg 2 (DOBDC) and Zn 2 (DOBDC) no worse than 0.02 Å for the calculated equilibrium geometries. The transferability is at no worse than 0.01 and 0.03 Å for the calculated geometry of the redox-suspect Fe 2 (DOBDC) and its superoxide adduct π-O 2 . The geometry of the DOBDC in σ -(O 2 ) 1− x agrees better (<0.05 Å) with that of the oxidized form of the DOBDC. The changes in the oxidation state of DOBDC are also characterized by shifts in the frequencies of the vibrational modes. The C 1 –C 2 and C 1 –C 3 stretches must shift redwards as the bond orders decrease while the C 1 –O′ and C 2 –C 3 stretches must shift bluewards as the bond orders increase from the quinolate to the semiquinone forms of DOBDC. Reference [28] 28 establishes a degree of transferability of the deformation modes in the IR spectrum of the benzene ring of the free DOBDC to the IR spectrum of Ni 2 (DOBDC), a homologue of Fe 2 (DOBDC). As Fig. 3 shows, characteristic shifts of the C 1 –C 2 and C 1 –C 3 stretches redwards as well as the C 2 –C 3 and C 1 –O′ stretches bluewards in the IR spectra of the quinolate and semiquinone forms of DOBDC also do not support any significant changes in its oxidation state in Fe 2 (DOBDC) and π-O 2 . The experimental IR spectra of Fe 2 (DOBDC) and π-O 2 ( Fig. 3 ) in the frequency region occupied by the benzene ring modes correlate better with the computed IR spectrum of the quinolate form than with the computed spectrum of the semiquionone form of DOBDC. Although the experimental spectra show blue and red shifts from Fe 2 (DOBDC) to π-O 2 (1,130 to 1,124 cm −1 , 1,156 to 1,151 cm −1 , 1,188 to 1,197 cm −1 , 1,244 to 1,267 cm −1 ), which could by themselves signify oxidation of DOBDC, other and more drastic changes in the spectrum, which oxidation of the linker induces in the computed spectra ( Fig. 3 ) are mute in the experimental spectrum. Hence, this analysis by itself does not favour any significant change in the oxidation state of the ligand from Fe 2 (DOBDC) to π-O 2 . Thus, the trends in the band structure, geometry and vibrational spectroscopy suggest that the electronic structure is 1D during formation of π-O 2 . 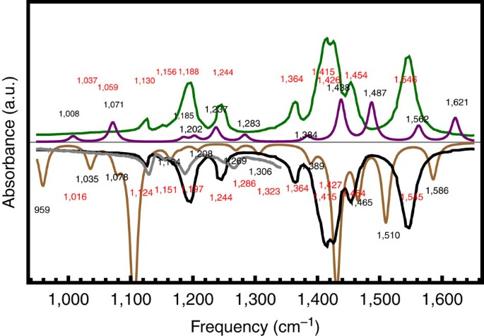Figure 3: The IR signatures of changes in the oxidation state in the MOF74. The experimental IR spectra from ref.9of Fe2(DOBDC) (green line), π-O2(grey line) andσ-O2(black line). The computed IR spectrum of the quinolate form of DOBDC (magenta line) and the semiquinone form of DOBDC (brown line). The red and black numbers label the experimental and computed absorption maxima, respectively. The absolute intensities of the transitions should not be compared between the different spectra. The IR-active modes at 1,621 cm−1(symmetric stretch along C1–C3), 1,562 cm−1(symmetric stretch along C1–C2), 1,487 cm−1(antisymmetric stretch along C1-C2), 1,438 cm−1(antisymmetic stretch along C1–C3) of the quinolate form shift to those at 1,389 cm−1(symmetric stretch along C1–C2), 1,306 cm−1(asymmetric stretch along C1–C2), 1,208 cm−1(asymmetric stretch along C1–C3), 1,180 cm−1(asymmetric stretch along C1–C3) of the semiquinone form. Meanwhile, the IR-active mode 1,283 cm−1(asymmetric C1–O′ and C2–C3stretches) in the quinolate form ends up at 1,431 cm−1in the semiquinone form. Figure 3: The IR signatures of changes in the oxidation state in the MOF74. The experimental IR spectra from ref. 9 of Fe 2 (DOBDC) (green line), π-O 2 (grey line) and σ -O 2 (black line). The computed IR spectrum of the quinolate form of DOBDC (magenta line) and the semiquinone form of DOBDC (brown line). The red and black numbers label the experimental and computed absorption maxima, respectively. The absolute intensities of the transitions should not be compared between the different spectra. The IR-active modes at 1,621 cm −1 (symmetric stretch along C 1 –C 3 ), 1,562 cm −1 (symmetric stretch along C 1 –C 2 ), 1,487 cm −1 (antisymmetric stretch along C 1 -C 2 ), 1,438 cm −1 (antisymmetic stretch along C 1 –C 3 ) of the quinolate form shift to those at 1,389 cm −1 (symmetric stretch along C 1 –C 2 ), 1,306 cm −1 (asymmetric stretch along C 1 –C 2 ), 1,208 cm −1 (asymmetric stretch along C 1 –C 3 ), 1,180 cm −1 (asymmetric stretch along C 1 –C 3 ) of the semiquinone form. Meanwhile, the IR-active mode 1,283 cm −1 (asymmetric C 1 –O′ and C 2 –C 3 stretches) in the quinolate form ends up at 1,431 cm −1 in the semiquinone form. Full size image Consequences of the electron flow being low dimensional To show that the consequences of the electronic structure being 1D are the anomalies observed in the O 2 adsorption experiments, a model is considered. Adsorbing O 2 applies the electron chemical potential at the exposed Fe sites to the electrons in the 1D bands Λ a 0 at the chemical potential μ e , so that O 2 acquires and the band Λ a 0 loses an average of electrons per site as the equilibrium condition requires. The lattice Hamiltonian of a three-band generalized Hubbard model [20] , describes the electrons within the triple of the bands Λ a 0 at a given or μ e in a finite chain of the Fe sites subject to the open boundary conditions at the left and right ends of the chain. Here, r =( λξ ) indexes the distinct Fe sites, λ =0, 1, 2 labels the translationally distinct sites within a unit cell (that are related by the third-order twist axis), while 0< ξ ≤ L /3 labels the unit cells in a chain of L Fe sites; t r 1 r 2 are the intersite hopping parameters; and U and V r 1 r 2 are the intra- and intersite electron-electron repulsion parameters, respectively. a r σ and are the Fermion creation and annihilation operators for the spin channels σ =↑,↓, and and n r = n r ↑ + n r ↓ . Then η r =2−‹ n r › is the quantum average and . The parameters in the Hamiltonian equation (1) are obtained from the PW91 band structure and the experimental UV/vis spectrum as detailed in Methods sections (Density functional theory calculations and Model of interacting electrons). As changes during O 2 adsorption, the charge distribution at a site r deviates from its average in a pattern telling of the mechanics of O 2 adsorption but also defined by the interaction between the electrons in a 1D partially filled band [20] . Since the latter cannot be disregarded, the problem of the electronic motion in the Λ a 0 bands belongs to a methodologically challenging domain, which, however, can be accessed numerically within the density matrix renormalization group [23] . The total energy, the electron chemical potential and the charge distribution η r for the ground and first excited states of the Hamiltonian equation (1) are computed for the chains of Fe sites at a conserved and even total number of the electrons using DMRG [23] as detailed in Methods section (DMRG calculations). To show that metal–insulator–metal transitions occur at about , , the charge excitation gap Δ≥0 is calculated using DMRG for a range of and U . Δ measures the minimal energy to displace the electrons. A partially filled ideal 1D conduction band can open a gap Δ>0 for the charge excitations so that the state of the electrons is insulating only at particular and rational fillings of the band; otherwise Δ=0 so that the state of the electrons is metallic (that is a Luttinger liquid) [20] . As shown in Fig. 4a , Δ peaks at about , , which corresponds to the insulating states. Lower values of Δ correspond to ‘metallic’ states. The charge compressibility (that is, the derivative of the volume of the electrons versus the chemical potential, Supplementary Fig. 3 ) diverges before the excitation gap opens, which further confirms that the gap openings are metal–insulator transitions. 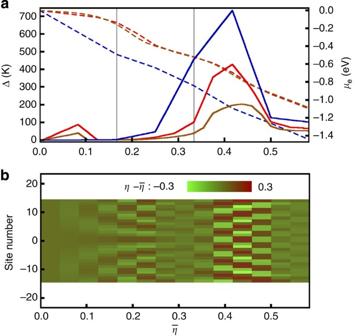Figure 4: Metal–insulator–metal transitions in the MOF74. (a) The charge gap Δ versus(solid lines) and the electron chemical potentialμeversus(dashed lines) forU=0.5 eV and for the chains of 24 (blue), 48 (red) and 96 (brown) Fe sites. (b) The ground state electron distributionversusand the site number for the chain of 48 Fe sites andU=0.5 eV. Figure 4: Metal–insulator–metal transitions in the MOF74. ( a ) The charge gap Δ versus (solid lines) and the electron chemical potential μ e versus (dashed lines) for U =0.5 eV and for the chains of 24 (blue), 48 (red) and 96 (brown) Fe sites. ( b ) The ground state electron distribution versus and the site number for the chain of 48 Fe sites and U =0.5 eV. Full size image To show that the process for a small enough δη >0 is activationless for or but the significant activation barrier of E ≠ =0.5Δ emerges near , it is sufficient to note that there have to be thermally accessible charge transfer excited states for the charge to flow to O 2 . The concentration of the thermally activated charge carriers scales as since the thermal excitations take place between the chemical potential level in the middle of the gap (up to the accuracy logarithmic in T ) and the states at the energies above Δ. Defects in the distribution of O 2 in π-O 2(1− x ) set a finite length scale above which ideal chains of Fe sites terminate. The gap Δ decreases towards its asymptotic value as the length increases. At the U =0.5 eV, E ≠ are 367, 214, 101 K for the chains of 24, 48, 96 Fe sites at , respectively. This temperature range is consistent with the empirical T A of 220 K. To explore the sensitivity of the model equation (1) on the parameter U , Fig. 5 compares the computed charge gaps. Although the magnitude of the gap (and T A ) depends on U , the fractional filling of the conduction band at which the metal–insulator–metal transition occurs is independent of . Therefore, the qualitative conclusions about O 2 adsorption driving the metal–insulator–metal transition still stand even if U , which enters equation (1), were in error or assumed a range. 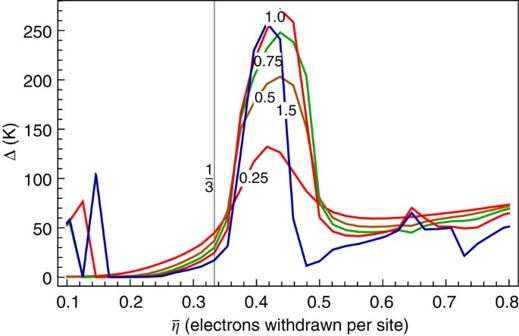Figure 5 The charge gap Δ versusfor a range ofUfor the chain of 96 Fe sites. Figure 5 The charge gap Δ versus for a range of U for the chain of 96 Fe sites. Full size image To show that a pronounced pattern of Fe II -like and Fe III -like sites emerges past the metal–insulator–metal transition at around , the distribution is computed ( Fig. 4b ). In the ‘metals’, η r exhibits a charge density wave modulation whose period is incommensurate with the lattice, the cost for displacing a charge Δ ≈0, and all Fe sites are nearly equivalent in a finite chain. However, the ground-state η r ( Fig. 4b ) exhibits charge density wave modulation, whose period is commensurate with the lattice of Fe sites in the insulating state near where the cost for displacing the charge is finite. Therefore, the maxima and minima of η r follow the Fe sites for , and the amplitude of the charge oscillations reaches about 0.6 e. For the insulator metallizes once again, but the modulation at around defines the new periodic background for the remaining electrons. A mechanism of adsorption of O 2 in Fe 2 (DOBDC) is now manifest. The initial O 2 adsorption triggers the insulator–metal transition above the O 2 coverage at which the applied electron chemical potential due to O 2 exceeds the gap in the correlated semiconductor Fe 2 (DOBDC) [20] . The minimum work to desorb η electrons from to Λ a 0 is − μ e η . If the work, kT , due to pressure change from P 0 to P 1 can overcome μ e η , then O 2 adsorption is reversible. μ e changes slowly with in the metallic state for where the charge distribution remains homogeneous in average. However, μ e jumps to a lower value past the metal–insulator–metal transition because of the stabilization of the pattern of the distinct sites, and with η r ′ < η r ′′ , which minimizes the electron repulsion. If , the activation barrier hinders the metal–insulator–metal transition at , and the O 2 adsorption halts at . In contrast, if , the charge transfer to O 2 proceeds to where the pattern of weaker and stronger bound emerges, O 2 desorbs from but remains at . The further pumps the electrons and converts to σ-O 2 while the DOBDC partially oxidizes. This mechanism implies further observable consequences. The optical conductivity σ ( ω ) of Fe 2 (DOBDC)+O 2 must be suppressed at the frequencies , but at it should show a scaling law σ ( ω ) ∝ (Δ− ω ) 3 K −4 where the exponent is determined by the Luttinger liquid parameter characteristic of a 1D system [20] . Conversion of the weakly bound π-O 2 to strongly bound σ-O 2 is undesirable in the context of the separation. If the mechanism is correct, the conversion is an activated process whose rate should decrease if the length of Fe chains unterminated by defects is decreased or if the electron repulsion U at Fe sites is changed ( Fig. 4a ; Supplementary Fig. 4 ), given that all other factors are fixed. Unlike non-porous low-dimensional materials, whose electronic structure is accessed by penetrating radiation at long range, the nano-porous materials offer the unique advantage that their geometry and long-range electronic structure can also be accessible at short range through by a more diverse probe: a chemical reaction. This report shows how O 2 chemisorption, a probe reaction, reflects the profound changes in the electronic structure throughout the material. Chemistry of electron acceptors other than O 2 in Fe 2 (DOBDC) can be similarly anomalous. Many heterogeneous catalytic reactions are redox processes [1] . If an electronically 1D MOF is a catalyst, then its chemical profile is likely anomalous. The material Fe 2 (DOBDC) belongs to a broader class of nano-porous materials whose geometry is 1D [29] . Those materials in this class, which are also electronically 1D, should exhibit anomalous chemical profiles, which may follow the pattern that is described in this report. The electronic structure of a nano-porous material may further delocalize and become two dimensional if the linkers become conductors. By tailoring the geometry of the electronic distribution through varying the chemistry of the charge transfer network in a MOF and adjusting external conditions, the chemistry of the material could be modulated. Density functional theory calculations The initial magnetic structure of Fe 2 (DOBDC) in the self-consistent DFT calculations is taken to be consistent with the magnetic susceptibility measurements [7] , [9] , which point to the magnetic order such that the spin 2 magnetic moments at Fe sites are parallel within a helical Fe chain and are antiparallel in the helical chains of the opposite chirality. The spin-orbit coupling is neglected. The geometries of Fe 2 (DOBDC) and π-O 2 are obtained by minimizing the total ground state energy with respect to the atomic displacements. The residual total force and the stress at the optimized geometries are below 0.1 eV·Å −1 and 1·10 −4 eV·Å −3 , respectively. The term ‘band structure’ denotes here the spin-unrestricted mean field PW91+U band structure. The PW91+U mean field model corrects the Perdew-Wang 91 (PW91) generalized gradient approximation (that is, PW91+U at U =0) for the underestimation of the Hubbard repulsion U >0 between the strongly correlated d -electrons at Fe sites. The value of U is set by the condition that the experimental and computed band gaps match ( Supplementary Fig. 1 ). The mean field of the ultrasoft pseudopotentials [21] replaces the electrons in the ionic cores Fe[Ne], C[He], C[He] and H. The Kohn-Sham Bloch wavefunctions and the electron densities of the remaining electrons are then expanded into the Fourier series up to the plane wave kinetic energy cutoffs of 476.2 and 5,714.4 eV, respectively. The numerical integration over the reciprocal space is carried over 1 a × 1 b × 4 c Monkhorst-Pack quadratures in the total energy and geometry optimization calculations. In the band structure calculations, the reciprocal space integration is carried over the 4 a × 4 b × 8 c , and then over the 1 a × 1 b × 71 c Monkhorst-Pack grids, after it is determined that the dispersion in the ab directions is much smaller than that along the c direction. The Gaussian occupation number smearing of 0.136 eV is applied when the band structure is metallic. The projected densities of states are computed with respect to the projections on the valence states of the atoms. Equilibrium geometry and vibrational frequencies of the ligand The equilibrium geometries and harmonic vibrational frequencies for the quinolate and semiquinone forms of the DOBDC are computed using the PW91 approximation to the exchange-correlation energy as implemented in ref. 22. The Kohn-Sham orbitals are expanded over the Pople’s gaussian basis set 6−311++ G (3 df , 3 pd ). The numerical integration in the exchange-correlation contributions to the energy, forces and frequencies is carried over atomic-centred Euler-Lebedev quadratures with 99 × 590 points along the radial and the angular directions per atom, respectively. The maximum forces at the equilibrium structures do not exceed 10 −3 eV·Å −1 . Crystal field Hamiltonian: top-down approach The ground state configurations of the free isotropic ion Fe 2+ is 3 d 6 . The electron–electron interaction arranges 210 degenerate states of the 3 d 6 configuration into 16 multiplets [19] . The restriction of the Hamiltonian onto the Hilbert space spanned by the multiplets of the configuration 3 d 6 (ref. 30 ) is The two-particle Hamiltonian acts on the states of the configuration 3 d 6 as where the Slater-Condon parameters [31] , , and set the strength of the electron–electron interaction. The H ee is block diagonal in the basis | LM L SM S ι › of the eigenstates of the total orbital and electronic spin angular momenta operators L 2 , L 3 , S 2 and S 3 ; the quantum number ι discriminates the terms of identical L and S in the configuration. The crystal field operator contains only the s -, d -, h -moments, , in its multipole expansion at an Fe site, The matrix elements of the unit spherical tensors are computed standardly [30] . For the purpose of the phenomenological analysis, the crystal field spherical moments are written in the form where R A and n A are the radius of the sphere centered at Fe 0 , and the position at this sphere of an ion A in the crystal structure, Y l , q are the surface spherical harmonics. Effective charges Z A are computed using the Bader population analysis [32] . The phenomenological parameters ρ 2 , ρ 4 , are constrained by the experimental UV/vis absorption spectrum of ref. 9 . First, the parameters ρ 2 , ρ 4 are found by the minimization of the least-square deviation between the spectrum of the crystal-field Hamiltonian and the transitions in the UV/vis absorption spectrum. Second, starting from the Hamiltonian at the optimal ρ 2 and ρ 4 , the eight independent parameters and are determined. Thus, determined the real and the imaginary parts of the parameters are The real and the imaginary parts of thus determined Hamiltonian in the basis |2 M L 200› for M L = −2, −1, 0, 1, 2 are and The angular distributions, of the electrons at an Fe site in the crystal field states are then defined by the eigenvectors c m ( 5 A 0,1,2,3,4 ) of the crystal field Hamiltonian in the basis of the d -orbitals. Crystal field Hamiltonian: bottom-up approach To further corroborate the phenomenological picture and establish the electronic distribution in the low-lying electronic states, the low-lying excited states of Fe 2+ and [Fe−O 2 ] 2+ are computed in the CIS(D), and state-averaged CASSCF MP2 approximations, as well as using the linear response time-dependent density functional theory in the adiabatic PW91 approximation. The molecular orbitals in these methods are expanded over the Dunning basis set aug — cc — pvtz of Gaussian functions as implemented in ref. 22. The single-particle external potential, represents the crystal field that the Fe site experiences; here the summation runs over the scaled Bader charges λ CF Z A of the ions within the ball centred at Fe site of the 60 Bohr radius; the screening exponent α is 0.035 Bohr −1 . The external potential is taken the same in the Fe 2 (DOBDC) and in π-O 2 at a vanishingly small O 2 load. The reference in the CIS(D) approximations is a stable unrestricted Hartree-Fock determinant. The initial orbitals that generate the active space in the CASSCF and CASSCF MP2 methods are the natural orbitals of the unrestricted Hartree-Fock density matrix. The six-electron active space of the Fe 2+ ion includes the five a 0 , a 1 , a 2 , a 3 , a 4 3 d -like orbitals. The eight-electron active space of the [Fe−O 2 ] 2+ includes seven orbitals that arise from the a 0 , a 1 , a 2 , a 3 , a 4 orbitals of the Fe 2+ and the two 1π g -like orbitals of O 2 . Model of interacting electrons The kinetic energy matrix of the three-band model is and its Fourier transform is the kinetic energy in the reciprocal space, The parameters ?, t 1 , t 2 , t 3 are obtained by matching the PW91 GGA band structure along the direction Z ΛΓΛ Z ( Supplementary Fig. 5 ) to the three independent unitary invariants of the 3 × 3 matrix, which are taken as the trace, the trace of the square, and the determinant, Thus determined hopping matrix elements are listed in Table 3 . The interaction is taken to be given by the Ohno–Klopman extrapolation formula, Table 3 Hopping matrix elements (in meV) for Fe 2 (DOBDC) at the geometry of π -O 2 . Full size table where the on-site electron repulsion is U , and a 0 is the Bohr radius. On the lattice, the distances between the 1 · Fe and 3 + · Fe, , sites are R 12 =3.2 , R 13 =5.2, R 14 =7.1 Å, respectively. The exponential screening at the length scale of l , no matter how long, in the bulk material, ensures that the Coulomb interaction is short range in the macroscopic limit; l is set to R 14 here. The exchange integrals, which are much smaller than the Coulomb integrals in the atomic case [31] , are neglected. DMRG calculations The total energies and the charge distribution in the ground and low-lying excited states of the model equation (1) are computed using DMRG approach. The maximum number of the states spanning the DMRG Hilbert space is increased from the initial 20 to 200 in six sweeps. The truncation errors do not exceed 10 −7 eV. The ground state at conserved N and L includes the total spin S =0 state. The gaps between excited states at given L and N are then determined by computing the ground and the first excited states at fixed S =0, 1 and N . The derivatives of the ground state energy in the expression of the chemical potential, and the charge compressibility, are computed numerically, at a given L . How to cite this article: Maximoff, S. N. and Smit, B. Redox chemistry and metal–insulator transitions intertwined in a nano-porous material. Nat. Commun. 5:4032 doi: 10.1038/ncomms5032 (2014).